Enhanced meta-analysis and replication studies identify five new psoriasis susceptibility loci Psoriasis is a chronic autoimmune disease with complex genetic architecture. Previous genome-wide association studies (GWAS) and a recent meta-analysis using Immunochip data have uncovered 36 susceptibility loci. Here, we extend our previous meta-analysis of European ancestry by refined genotype calling and imputation and by the addition of 5,033 cases and 5,707 controls. The combined analysis, consisting of over 15,000 cases and 27,000 controls, identifies five new psoriasis susceptibility loci at genome-wide significance ( P <5 × 10 −8 ). The newly identified signals include two that reside in intergenic regions (1q31.1 and 5p13.1) and three residing near PLCL2 (3p24.3), NFKBIZ (3q12.3) and CAMK2G (10q22.2). We further demonstrate that NFKBIZ is a TRAF3IP2 -dependent target of IL-17 signalling in human skin keratinocytes, thereby functionally linking two strong candidate genes. These results further integrate the genetics and immunology of psoriasis, suggesting new avenues for functional analysis and improved therapies. Psoriasis is a chronic immune-mediated skin disease with complex genetic architecture that affects ∼ 2% of the world population. It presents a significant economic burden for affected individuals and for society [1] , and can severely impact the patient’s quality of life [2] . Aided by advances in high-throughput genotyping technologies, genome-wide association studies have identified multiple genetic loci associated with psoriasis [3] , [4] , [5] , [6] . These studies have been accompanied by replication of the most promising signals to confirm the psoriasis-associated signals at genome-wide significance levels. More recently, large consortia have utilized meta-analyses to identify additional susceptibility loci with modest effect sizes [7] , [8] . Previously, we performed a meta-analysis combining three existing GWAS [the Collaborative Association Study of Psoriasis (CASP) [3] , Kiel [5] , the Wellcome Trust Case Control Consortium 2 (WTCCC2) [6] and two Immunochip data sets (the Genetic Analysis of Psoriasis Consortium (GAPC) and the Psoriasis Association Genetics Extension (PAGE))) and identified 15 novel psoriasis susceptibility loci [8] , increasing the number of confirmed loci to 36 for populations of European descent. In this study, we enhanced our previous meta-analysis [8] and added replication data sets to follow up the most promising signals. First, we applied the optiCall [9] genotype calling algorithm to the GAPC and PAGE data sets, and performed genome-wide imputation to 1,000 Genomes haplotypes. In this way, we were able to examine association at over six times the number of variants examined in our previous meta-analysis [8] . Using these enhancements, we perform a discovery meta-analysis of the combined GAPC/PAGE Immunochip data set and the three psoriasis GWAS [3] , [5] , [6] , [7] , comprising 10,262 psoriasis cases and 21,871 controls. We then conduct replication analysis in 5,033 cases and 5,707 controls from four independent data sets, resulting in a combined analysis involving over 15,000 cases and 27,000 controls. We report five novel psoriasis susceptibility loci reaching genome-wide significance ( P <5 × 10 −8 ), which add to the collective understanding of the genetic basis of this common cutaneous disorder. Discovery meta-analysis The discovery meta-analysis included the combined GAPC/PAGE Immunochip data set and three existing GWAS data sets (that is, CASP, Kiel and WTCCC2). We first performed genome-wide imputation of each data set using 1000 Genomes haplotypes as a reference panel [10] . After imputation, we tested association for 696,365 markers (52,444 of them are short insertion/deletion variations, INDELs) that had minor allele frequencies (MAF) ≥1% and imputation quality ( r 2 ) >0.7 in all the four data sets. This study analysed more than six times the 111,236 markers examined in the original meta-analysis [8] . We have shown that linear mixed modelling could be used to correct population stratification for association analysis [11] in the PAGE and GAPC data sets separately [8] . This is also the case in the current combined Immunochip data set consisting of 6,268 psoriasis cases and 14,172 controls, with the genomic inflation factor estimated to be 0.96 ( Supplementary Fig. 1 ). The genomic inflation factors for the CASP, Kiel and WTCCC2 GWAS data were estimated to be 1.01, 1.04 and 1.04, respectively. Among the 36 known psoriasis susceptibility loci, 35 yielded strong evidence of association (effective sample-size weighted z -score: P discovery-meta ≤5 × 10 −7 ), of which 30 achieved genome-wide significance ( P discovery-meta ≤5 × 10 −8 ) in the discovery meta-analysis ( Supplementary Information and Supplementary Fig. 2 ) involving 10,262 cases and 21,871 controls. The only previously described locus that did not yield association in this study maps near IL28RA , in which the strongest previously identified signals [6] failed our quality filters in one of the GWAS data sets. However, the Immunochip data alone does show suggestive association in the IL28RA region (EMMAX: P Immunochip =3.5 × 10 −7 ). 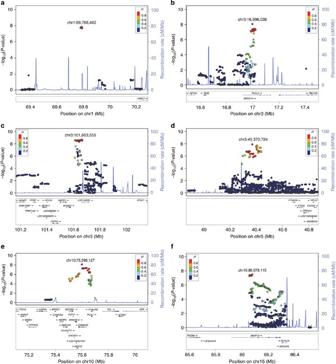Figure 1: Regional association plots for novel psoriasis susceptibility loci. (a–f) This figure depicts LocusZoom-generated association plots for the six psoriasis susceptibility loci identified in the discovery meta-analysis (effective sample-size weighted approach). All but the 15q25.3 locus (f) showed genome-wide significant results in the combined meta-analysis. Combined analysis identifies five new loci In the discovery meta-analysis, we identified six novel loci showing significant association with P discovery-meta ≤5 × 10 −8 ( Table 1 , Fig. 1 and Supplementary Table 1 ). 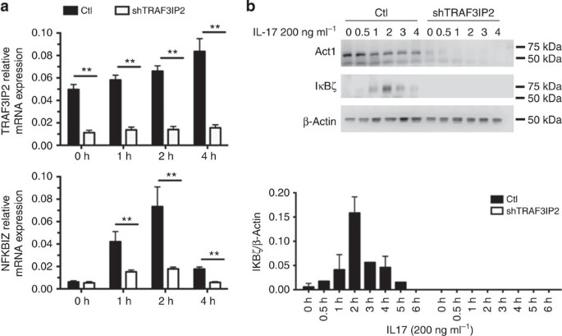Figure 2:NFKBIZmRNA and IκB-zeta protein are induced by IL-17 in an Act1-dependent fashion in human keratinocytes. (a) Time courses ofTRAF3IP2(top) andNFKBIZ(bottom) mRNA expression following IL-17 induction. Black bars represent mRNA relative expression levels measured by qPCR in the absence of tetracyline (Tet) while white bars represent levels after silencingTRAF3IP2expression via Tet-inducible expression of shTRAF3IP2. Bars are mean+s.e.m. of three independent experiments and **P<0.01; Student’st-test. (b) Western blot analysis of time courses of IκB-zeta and Act1 expression (upper panel) and quantifications of IκB-zeta band intensity relative to β-actin. Bars are mean+s.d. of two independent experiments (lower panel). We evaluated the most strongly associated markers (that is, the ‘best markers’) identified in the new loci, and all of them have good imputation quality and none exhibited significant heterogeneity across data sets (all heterogeneity P -values>0.1; Supplementary Table 2 ). We then expanded our analysis utilizing genotyping data from four independent replication data sets, utilizing either the best markers or their best linkage disequilibrium (LD) proxies if LD- r 2 ≥0.8. Notably, five of the six loci retained genome-wide significance in the combined meta-analysis ( Table 2 ; Supplementary Table 3 ). Because one of the best markers (rs4685408) was genotyped separately in a substantial fraction (3,030 cases and 2,859 controls) of two of our replication data sets (that is, Exomechip 2 and PsA GWAS; Table 2 ), and the proxies for this marker in the two data sets were among the weakest of those listed in Table 2 , we also treated this data as an additional independent data set (termed as ‘Michigan Genotyping’ in Supplementary Table 3 ; logistic regression: P Michigan =9 × 10 −5 ; combined meta-analysis: P combined-meta =9 × 10 −15 ). In all, the combined analysis consists of around 15,000 psoriasis cases and over 27,000 controls. Table 1 Loci with genome-wide association signals identified in the discovery meta-analysis. Full size table Figure 1: Regional association plots for novel psoriasis susceptibility loci. ( a – f ) This figure depicts LocusZoom-generated association plots for the six psoriasis susceptibility loci identified in the discovery meta-analysis (effective sample-size weighted approach). All but the 15q25.3 locus ( f ) showed genome-wide significant results in the combined meta-analysis. Full size image Table 2 Results from the discovery, replication and combined meta-analysis. Full size table The estimated odds ratios (ORs) for the five confirmed novel loci ranged from 1.12 to 1.17 ( Table 1 ), similar to the 15 new loci identified in the original meta-analysis [8] . Among the five novel loci, 5q13.1 has the highest effect size (OR=1.17). Interestingly, this signal is situated in an intergenic region ( Fig. 1 ), and was previously identified as a susceptibility locus for other autoimmune diseases including inflammatory bowel disease and multiple sclerosis ( Table 3 ). While additional comparisons and more well-powered studies are needed, none of the five novel loci reported here have been identified as genome-wide psoriasis susceptibility loci in non-European samples [4] , [12] , [13] , [14] , [15] ( Supplementary Table 4 ). Table 3 Newly discovered psoriasis loci that are shared with other disease susceptibility loci according to NHGRI GWAS catalogue. Full size table As assessed using ANNOVAR [16] , the strongest signals from three of the confirmed loci map to intronic regions ( Table 1 ), and the strongest signals from the other two loci map to intergenic regions. Using 1000 Genomes Project data, we did not identify any common (MAF>1%) protein-altering variants (that is, missense/nonsense mutations) in high LD (LD- r 2 ≥0.8) with our strongest signals. We also performed conditional and interaction analyses using the five new loci identified in this study and did not identify any independent secondary signals within the five loci or evidence for epistasis effects among these loci or with previously described psoriasis loci. Biological inferences for identified loci Nearby genes within the three non-intergenic susceptibility loci (within ±200 kb boundary of the strongest signals) include: PLCL2 on 3p24.3; NFKBIZ, ZPLD1 and CEP97 on 3q12.3; and CAMK2G , FUT11, AGAP5 , PLAU and MYOZ1 on 10q22.2 ( Fig. 1 ). Among the above genes, NFKBIZ and MYOZ1 were differentially expressed when comparing psoriatic and normal skin samples [17] : NFKBIZ was 4-fold up-regulated (Wilcoxon rank-sum test: P= 1.1 × 10 −28 ) and MYOZ1 was down-regulated (fold change=0.5; P= 3.5 × 10 −14 ) in lesional psoriatic skin versus normal skin. We searched the NHGRI catalogue [18] for previously identified genome-wide significant ( P ≤5 × 10 −8 ) loci within ±200 kb of the best signals from the five novel loci identified in this study. Four of the five new loci are shared with other complex traits, most of which are immune-mediated inflammatory disorders ( Table 3 ). For the most part, however, the risk variants from psoriasis and the other complex traits that map to the same loci are not in LD, meaning that the psoriasis risk haplotypes do not tend to be the same as those found for the other traits ( Table 3 ). Although intergenic in nature, the 5p13.1 locus is shared with four other complex diseases, including allergy [19] , multiple sclerosis [20] , Crohn’s disease [21] , [22] and ulcerative colitis [23] . As the novel signals do not tend to be in LD with any amino-acid altering variants, we then investigated their potential regulatory roles. Of the five novel loci, four of them overlapped with histone marks or transcription factor binding sites in lymphoblastoid cells or keratinocytes according to data from ENCODE [24] ( Supplementary Table 5 ). The transcription factors (for example, NF-κB, IRF4, BATF, JUN-D) for the binding sites overlapped by these loci tend to be involved in immune responses: NF-κB and IRF4 are important transcription factors that regulate both innate and adaptive immune response; and the BATF–JUN family protein complexes are essential for IRF4-mediated transcription in T cells [25] . We then asked whether our best markers from the novel loci are eQTLs and could alter the expression of nearby genes. Interestingly, we found that rs7637230 ( P =2.22 × 10 −8 ) and rs2675662 ( P =5.78 × 10 −10 ) are both cis-eQTLs in lymphoblastoid cells [26] , and affect the expression levels of NFKBIZ and FUT11 , respectively. The IL-17 pathway has been shown to play an important role in psoriasis [27] . TRAF3IP2 , a susceptibility locus for both psoriasis and psoriatic arthritis [5] , [8] , [28] , encodes adaptor protein Act1, one of the key components in the IL-17 signalling pathway [29] . NFKBIZ , a gene in one of the newly discovered loci of this study, has been shown to be an Act1-dependent IL-17 target gene in mice [30] , [31] . Because psoriasis is a uniquely human disease, and because keratinocytes appear to be a key target of IL-17 action in psoriasis [27] , we set out to determine whether NFKBIZ is also an Act1-dependent target of IL-17 signalling in human keratinocytes. To do this, we investigated the time course of NFKBIZ expression in human keratinocytes engineered to silence TRAF3IP2 expression under the control of tetracycline. As shown in Fig. 2 , expression of NFKBIZ mRNA and protein could be significantly induced by IL-17 ( P <0.01), and these inductions were significantly ( P <0.01) blocked by TRAF3IP2 silencing. As illustrated above, variant rs7637230 is in strong LD ( r 2 ≥0.8) with markers that overlap with chromatin marks in lymphoblastoid cells and keratinocytes ( Supplementary Table 5 ) and it is an eQTL for the expression of NFKBIZ in lymphoblastoid cells [26] . Together with the results from our NFKBIZ experiments, these findings nominate NFKBIZ as a strong candidate gene in the 3q12 locus and suggest a potential disease mechanism of the IL-17 pathway in psoriasis. Figure 2: NFKBIZ mRNA and IκB-zeta protein are induced by IL-17 in an Act1-dependent fashion in human keratinocytes. ( a ) Time courses of TRAF3IP2 (top) and NFKBIZ (bottom) mRNA expression following IL-17 induction. Black bars represent mRNA relative expression levels measured by qPCR in the absence of tetracyline (Tet) while white bars represent levels after silencing TRAF3IP2 expression via Tet-inducible expression of shTRAF3IP2. Bars are mean+s.e.m. of three independent experiments and ** P <0.01; Student’s t -test. ( b ) Western blot analysis of time courses of IκB-zeta and Act1 expression (upper panel) and quantifications of IκB-zeta band intensity relative to β-actin. Bars are mean+s.d. of two independent experiments (lower panel). Full size image In this study, we identified five novel psoriasis susceptibility loci reaching genome-wide significance, increasing the number of known psoriasis susceptibility loci to 41 in Caucasians and to 49 worldwide ( Supplementary Table 4 ). We performed three main procedures to ensure the validity of the identified novel loci in this study: First, to ensure that the imputed dosage of each marker is accurate and to avoid batch effects, we required a stringent imputation quality threshold ( r 2 ≥0.7). Furthermore, we only considered markers that passed the quality threshold in all the four data sets when performing the associations ( Supplementary Table 2 ). Second, we calculated the heterogeneity P -value from the meta-analysis to be sure that the associations were not heterogeneous ( P >0.05) among the data sets ( Supplementary Table 2 ). Finally, we performed a replication analysis to further validate that the 5 loci still achieve genome-wide significance in the combined meta-analysis ( Table 2 ). Although estimates of allele frequencies based on imputed dosages will have added uncertainty compared with those based on experimentally determined genotypes, the allele frequencies reported in our study do show consistent differences between cases and controls for each of the associated markers across different data sets ( Supplementary Table 2 ). We also compared risk allele frequencies for 41 psoriasis susceptibility loci across the four discovery data sets, and we observed very high concordance ( r 2 ≥0.99) of the estimated frequencies in controls for all six possible pairs of data sets ( Supplementary Fig. 3 ). Three of the five newly identified loci contained protein-coding genes; however, we found no evidence suggesting that our signals are missense or nonsense mutations, nor are they in LD with such variations. Our results are in agreement with data for other known psoriasis susceptibility loci, in that fewer than 25% of the psoriasis-associated signals are in LD with codon-changing variations [8] . Although no deleterious functional variants were identified in the three protein-coding loci ( PLCL2 at 3p24.3; NFKBIZ, ZPLD1 and CEP97 at 3q12.3; and CAMK2G , FUT11, AGAP5 , PLAU and MYOZ1 at 10q22.2), variation in PLCL2 has previously been shown to be associated at genome-wide significance ( P =2.3 × 10 −8 ) with primary biliary cirrhosis [32] and nominally ( P =1.7 × 10 −3 ) in a cohort of 982 Caucasian cases of psoriatic arthritis and 8,676 Caucasian controls [33] . In mice, NFKBIZ deletion has been functionally associated with inflammatory skin eruptions [34] and CAMK2G has been functionally implicated in thymic development [35] . In addition, PLAU , encoding urokinase-type plasminogen activator, has been reported to be overexpressed in psoriatic skin [36] and was up-regulated 1.49-fold ( P =3.7 × 10 −13 ) in our psoriasis RNA-seq transcriptome data, albeit short of the 2-fold change threshold we used to declare significance [17] . Of the remaining protein-coding genes in these three loci, MYOZ1 encodes myozenin, a muscle protein of no obvious relevance to psoriasis, and very little information is available for ZPLD1, CEP97 and AGAP5 in Online Mendelian Inheritance in Man [37] . The identification of the disease-associated single-nucleotide polymorphisms (SNPs) rs7637230 ( P =2.22 × 10 −8 ) and rs2675662 ( P =5.78 × 10 −10 ) as cis-eQTLs in lymphoblastoid cells [26] prioritizes NFKBIZ and FUT11 as strong candidate genes in their respective loci. Several recent clinical studies have shown benefit of blockade of IL-17 and its receptors in psoriasis [38] . In this context, the connection between NFKBIZ and TRAF3IP2 is of biological and therapeutic interest . TRAF3IP2 encodes Act1 (also known as CIKS), an ubiquitin ligase that binds to IL-17 receptors [39] , [40] . NFKBIZ encodes IκB-zeta, a transcriptional regulator that binds to the p50 subunit of NF-kB [41] . Act1 and IκB-zeta are required for IL-17-dependent signalling associated with autoimmune and inflammatory diseases [42] , [43] . Nfkbiz -deficient mice manifest defective Th17 development, and IκB-zeta regulates this process by cooperating with ROR nuclear receptors [43] . While Act1 has previously been shown to regulate Nfkbiz expression in mouse embryonic fibroblasts [30] and mouse skin keratinocytes [31] , this is the first demonstration of Act1-dependent NFKBIZ /IκB-zeta expression in human keratinocytes. Interestingly, TNFAIP3 encoding A20 is also a strong candidate gene in psoriasis and several other inflammatory diseases, which appears to act as a brake on cytokine-medicated signalling [44] . Interestingly TNFAIP3 is also an Act1-dependent target of IL-17 signalling, which, in turn, functions as a negative regulator of IL-17 receptor function [29] . These results highlight NFKBIZ as an IL17 target and identify an immunoregulatory network downstream of the IL-17 receptor involving at least three psoriasis candidate genes: TRAF3IP2 , NFKBIZ and TNFAIP3 . Evidence is accumulating to indicate that genetic variants in regulatory regions may play important biological roles in complex genetic disorders [45] , [46] , and large scale projects such as ENCODE [24] have been using sequencing technologies and integrative approaches to illuminate the functional elements of the human genome. Our results illustrate the potential regulatory roles of the psoriasis susceptibility loci, and will facilitate the design of future functional analyses. Similar to other complex traits and diseases [47] , [48] , large inter-continental consortia have been forming to gather hundreds of thousands of samples to identify susceptibility loci with very mild effect sizes for psoriasis. Moreover, the study of psoriasis genetics is entering a new era, with more efforts on investigating the missing heritability explained by secondary independent signals (fine-mapping analysis [49] , [50] ) and rare variants (by using exome-array or target-/exome-sequencing [15] ) in known loci. Not only will these studies provide a higher explained variance by the genetic components, more importantly, they will also shed light on the pathogenesis and disease mechanisms, and ultimately provide new approaches and targets for effective drug discovery. Discovery meta-analysis data sets Samples were collected at the participating institutions after obtaining informed consent, and enrolment of human subjects for this study was approved by the following ethics boards: UK samples—St Thomas' Hospital Research Ethics Committee; Estonian Biobank—Research Ethics Committee of the University of Tartu; Michigan samples—Institutional Review Board of the University of Michigan Medical School; German samples—Ethical review board of the Medical Faculty of the CAU (Christian-Albrechts-University of Kiel, Germany); Toronto samples—the ethics board is the University Health Network; Swedish samples—the ethics board is the Local Ethical Review Board at Linkóping University; Newfoundland samples—the ethics board is the Health Research Ethics Authority; Utah samples—the ethics board is the Institutional Review Board of the University of Utah. We first performed the discovery meta-analysis using four data sets: (i) combined GAPC/PAGE Immunochip data set; (ii) CASP GWAS; (iii) Kiel GWAS; and (iv) WTCCC2 GWAS. Since the algorithm implemented in optiCall, which uses both within- and across-sample signal intensities, can outperform standard methods (for example, GenCall or GenoSNP) [9] when applied to Immunochip, we used optiCall [9] to recall the PAGE and GAPC data sets. We removed samples with outlying intensity values based on optiCall default settings by using the ‘–meanintfilter’ flag. Samples with >2% missing genotypes and markers with >5% missing values were rejected. We merged the PAGE and GAPC data sets to form a unified Immunochip data set, re-applying the above call rate criteria to the combined data. These and subsequent genotype-dependent quality control procedures resulted in the removal of 1,222 (5.6%) samples from this analysis, compared with the previous study [8] . The quality-controlled Immunochip data set consisted of 2,858 cases and 8,636 controls in GAPC, and 3,410 cases and 5,536 controls in PAGE. For each of the three GWAS data sets, we first obtained the quality-controlled genotyped data used by the previous studies [3] , [5] , [6] . We then applied additional filters (sample/marker call rate ≥0.95; HWE P ≥1 × 10 −6 ) to the genotyped data before phasing/imputation (see below). Supplementary Table 6 shows the quality measurements for each data set. Imputation and association For each of the GWAS/Immunochip data sets, we performed haplotype phasing of the genotypes using ShapeIT [51] , we then performed imputation using minimac [52] using haplotypes from the EUR subset of version 3 of the 1000 Genomes Project Phase I release as the reference panel [10] . After imputation, we analysed markers with minor allele frequency (MAF) ≥1% and with imputation quality r 2 ≥0.7 in all the four data sets. For the Immunochip data, a linear mixed model was used to perform association tests as implemented in EMMAX [11] . The kinship matrix was computed using common (MAF>1%) independent markers located outside the 36 known psoriasis loci, having P GWA ≥0.5 (where P GWA represents the association P -values obtained from the meta-analysis using only the three independent GWAS data sets; this choice is common for analyses using ImmunoChip markers which are enriched for variants associated with psoriasis in our original GWAS). Using the same procedures described in the previous study for quality control [8] (that is, SNPs with call rate <95% or with a Hardy–Weinberg equilibrium P -value <1 × 10 −6 were excluded; samples with <95% call rate were excluded), we performed logistic regression on the three GWAS data sets (that is, CASP, Kiel and WTCCC2), using principal components as covariates to correct for population stratification [3] , [5] , [6] . Discovery meta-analysis We used METAL to perform meta-analysis, using the sample-size weighted approach [53] , adjusting the genomic control inflation factor separately for each data set. To estimate the odds ratios (ORs) for each marker, we first computed the ORs from the Immunochip data using logistic regression, and then used a sample-size weighted approach to compute the ORs from the full data sets [8] . The regional association plots were created by using the software LocusZoom [54] . We used ANNOVAR to perform variant annotations [16] using Gencode v19 (ref. 55 ) as gene references. Replication data sets and combined meta-analysis For each of the most strongly associated genome-wide significant ( P<5 × 10 − 8 ) markers (that is, the ‘best markers’) from the novel signals identified in the discovery meta-analysis, we used genotyping data obtained from four different collaborative data sets (here referred to as Exomechip 1, Exomechip 2, PsA GWAS and Genizon GWAS) for replication. If the best associated markers were not genotyped in the replication data sets, we identified the best proxies based on the LD (LD- r 2 ) in the European ancestry subset of version 3 of the 1000 Genomes Project Phase I release [10] . Only proxies with LD- r 2 ≥0.8 against our best signals were considered. Using only genetically independent samples, the 5,033 additional cases and 5,707 controls were combined with the discovery meta-analysis using the sample-size weighted approach [53] . NFKBIZ expression N/TERT-TR keratinocytes were engineered to express a tetracycline (Tet)-inducible shRNA as described [56] . These cells (N/TERT-TR-shTRAF3IP2) were seeded at 8,000 cells cm −2 in the presence or absence of 1 μg ml −1 Tet. When confluent (after 7 days), cells were stimulated for 1 to 4 h with 200 ng ml −1 recombinant human (rh) IL-17A (R&D Systems). RNA was isolated using RNAeasy columns (Qiagen) and reverse-transcribed using the High Capacity cDNA Reverse Transcription Kit (Life Technologies). Quantitative real-time polymerase chain reaction (qPCR) was performed using Taqman primers (Life Technologies) specific for nuclear factor of kappa light polypeptide gene enhancer in B-cells inhibitor, zeta ( NFKBIZ, Hs00230071-m1), TNF receptor associated factor 3 interacting protein 2 ( TRAF3IP2 , Hs00974570-m1) and the control gene RPLP0 ( Hs99999902_m1). From the same experiments, NFKBIZ and TRAF3IP2/Act1 proteins were assessed by western blotting, utilizing rabbit polyclonal IgG (respectively from Cell Signal Transduction #9244 and Santa Cruz Biotechnology sc-11444, both diluted 1:1,000) to detect protein, with β-actin (Cell Signal Transduction #4967 dilution 1:5,000) as a loading control. Statistical analysis was performed using GraphPad software (Prizm).The uncropped scans of the blots are shown in Supplementary Fig. 4 . Overlap with ENCODE genomic features We investigated whether the best signals identified from the novel loci are in LD with markers within chromatin marks or transcription factor binding sites. For each best associated marker, we first identified a set of high LD-markers based on the European population of the 1000 Genomes. We then examined human keratinocytes and lymphoblastoid cell lines (relevant cell types for psoriasis) and identified any chromatin marks or transcription factor binding sites overlapping with the LD-marks. How to cite this article: Tsoi, L. C. et al. Enhanced meta-analysis and replication studies identify five new psoriasis susceptibility loci. Nat. Commun. 6:7001 doi: 10.1038/ncomms8001 (2015).